A broad analysis of resistance development in the malaria parasite Microbial resistance to chemotherapy has caused countless deaths where malaria is endemic. Chemotherapy may fail either due to pre-existing resistance or evolution of drug-resistant parasites. Here we use a diverse set of antimalarial compounds to investigate the acquisition of drug resistance and the degree of cross-resistance against common resistance alleles. We assess cross-resistance using a set of 15 parasite lines carrying resistance-conferring alleles in pfatp4 , cytochrome bc 1 , pfcarl , pfdhod, pfcrt , pfmdr, pfdhfr, cytoplasmic prolyl t-RNA synthetase or hsp90 . Subsequently, we assess whether resistant parasites can be obtained after several rounds of drug selection. Twenty-three of the 48 in vitro selections result in resistant parasites, with time to resistance onset ranging from 15 to 300 days. Our data indicate that pre-existing resistance may not be a major hurdle for novel-target antimalarial candidates, and focusing our attention on fast-killing compounds may result in a slower onset of clinical resistance. Malaria remains a devastating disease, with an estimated 198 million cases (uncertainty range 124–283 million) and 584,000 deaths (uncertainty range 367,000–755,000) in 2013 alone, affecting primarily children under the age of five [1] . Given that the current vaccine available provides only moderate protection [2] , chemotherapeutics constitute the best clinical tools available for the prevention and treatment of malaria. Currently, A number of effective drug therapies exist, most of which target the malaria parasite during its replicative cycle within human erythrocytes, the lifecycle stage that is associated with clinical manifestations of malaria [3] . These consist of 4-aminoquinolines including chloroquine, piperaquine and related compounds; antifolates such as pyrimethamine and cycloguanil; alkanolamines such as halofantrine and lumefantrine; endoperoxides such as artesunate, artemisinin and artemether; and newer synthetic compounds. Antimalarial treatments are typically administered as combination therapies, and artemisinin-based combination therapies (ACTs, such as artemether-lumefantrine) currently represent the therapy class that is most effective and that is the standard of care recommended by the World Health Organization (WHO). While ACTs have been a highly effective frontline therapy, particularly against multidrug-resistant Plasmodium falciparum infections, there is now evidence of resistance emerging to artemisinin and its derivatives [4] , [5] , [6] , [7] . Clinical trials with artemisinin mono-therapies have shown that these compounds are taking considerably longer to clear malaria infections in Southeast Asia—typically twice as long as observed a decade ago. Given that parasites have already acquired resistance to several partner drugs, treatment failures are beginning to be observed with combination therapies [8] , [9] . Thus, new compound classes, ideally with new mechanisms of action, are urgently needed if the gains of the last decade are to be sustained. In anticipation of eventual widespread ACT failure, there has been a focused and coordinated effort to place new antimalarial drug candidates into the drug development pipeline (see http://www.mmv.org/research-development/rd-portfolio ). Leads from phenotypic screens in particular are being progressed into molecules that are suitable for testing in clinical trials. An open question, however, is whether small molecules from phenotypic screens will lead to the identification of new druggable targets and pathways that do not rapidly lose effectiveness in the field because of acquired and pre-existing parasite resistance. Here we use a set of 50 antimalarial compounds identified in phenotypic screens [10] , [11] , [12] , [13] to systematically evaluate whether resistant parasites can be selected and whether or not pre-existing resistance mechanisms confer resistance using a panel of strains containing mutations in a variety of genes, including P. falciparum cyclic amine resistance locus ( pfcarl) [14] , cytochrome bc1 (refs 15 , 16 , 17 ) and P. falciparum ATPase 4 ( pfatp4 ) [18] , [19] , [20] . Here we show that pre-existing resistance is less likely to be a problem but that the de novo acquisition of resistance occurs rapidly for many compounds. We highlight a set of antimalarial compounds that have thus far defied attempts to create drug-resistant parasites in a variety of different laboratories and identify features that are shared by all, including a rapid rate of killing and lack of pre-existing resistance. Initial selection of compounds To systematically investigate both the de novo acquisition and pre-existing landscape of drug resistance, we assembled a set of 50 diverse compounds selected from P. falciparum asexual phenotypic screens [10] , [11] , [12] , [13] . Compounds were initially chosen based on potency, demonstrated by activity against asexual blood stages ranging from 23 nM to 1.67 μM EC 50 with most compounds having an EC 50 of <1 μM in the P. falciparum strain 3D7 as measured by a hypoxanthine incorporation assay. To minimize non-novel pharmacophores, compounds were compared against the scaffolds of clinical antimalarials, eliminating candidates with similar structures. Compounds in our set ranged in molecular weight from 261 to 574 g·mol −1 , with 42 compounds having drug-like properties (compliant with Lipinski’s rule of five) and the remaining 8 identified as probe-like compounds. We sought to maximize chemical diversity in our set by eliminating similar compounds as indicated by the Tanimoto coefficient, since compounds with Tanimoto coefficients >0.85, a quantitative measurement of chemical scaffold similarity, are thought to have similar biological activity to one another [21] , [22] . The resulting compound set displayed an average Tanimoto coefficient of 0.186, ranging from 0.093 to 0.923 ( Fig. 1 ). Although a few compounds were similar to one another (particularly two carbazoles: MMV009063 and MMV665882) a majority of the set was diverse, possessing a variety of functional groups and heterocyclic substructures. 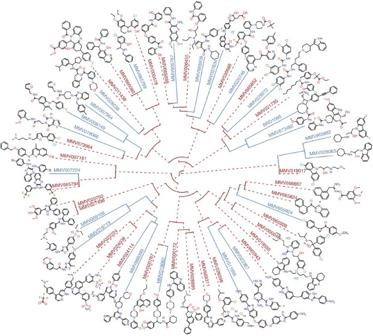Figure 1: Chemically diverse compound set. Hierarchical clustering of the 50 compound set. Compounds were clustered by a maximum substructure similarity Tanimoto coefficient.In vitroselections that were successful in yielding resistant parasites are highlighted in blue, whereas compounds where resistance development was unsuccessful are highlighted in dashed red. Figure 1: Chemically diverse compound set. Hierarchical clustering of the 50 compound set. Compounds were clustered by a maximum substructure similarity Tanimoto coefficient. In vitro selections that were successful in yielding resistant parasites are highlighted in blue, whereas compounds where resistance development was unsuccessful are highlighted in dashed red. Full size image Compound evaluation against a panel of resistant clones Multidrug resistance alleles, including mutations in P. falciparum chloroquine resistance transporter ( pfcrt) and P. falciparum multi-drug resistance transporter 1 ( pfmdr1 ) are very common in field isolates. Therefore, we sought to assess the degree to which pre-existing resistance alleles would contribute to a loss of potency for this diverse collection of small molecule compounds. Fifteen clones derived from three main parent lines were chosen to maximize diversity in mutated pathways and genetic backgrounds, thus representing the variety of resistance seen in the field: 3D7 (ref. 23 ), W2 (ref. 24 ) or Dd2 (ref. 25 ). The 3D7 line originates from the clone of a Netherlands clinical isolate strain [23] , [26] and is generally considered to be drug sensitive, though it does convey resistance to sulfadoxine. Conversely, W2 (ref. 24 , 27 ) and Dd2 (ref. 25 ) are multi-drug-resistant lines originating from the Indochina III/CDC isolate, which contain point mutations in pfcrt as well as amplifications in pfmdr1 and GTP cyclohydrolase [27] . A total of nine known drug-resistance genes were represented by our strain set, containing validated critical single nucleotide variants (SNVs) or copy number variants as well as a handful of additional background mutations. One strain, TM90C2A, was a clinical isolate from Thailand [28] , while the remaining 15 lines were created through in vitro evolution. Clones contained one or more resistance-conferring alleles in the folate pathway [28] , pfcrt (ref. 29 ), P. falciparum dihydroorotate dehydrogenase ( pfdhodh ) [30] , pfcarl (ref. 14 ), prolyl t-RNA synthetase [31] or heat shock protein 90 ( hsp90 ). We also investigated multiple cytochrome bc 1 (refs 15 , 16 , 17 ) and pfatp4 (refs 18 , 19 , 20 ) alleles, including three alleles in the cytochrome bc 1 Q o site, which confer resistance to atovaquone [15] or a tetracyclic benzothiazepine [16] and one allele in the cytochrome bc 1 Q i site conferring resistance to a benzylsulfonamide [17] . The five PfATP4 mutant lines possess alleles that map to the transmembrane channel of the sodium-dependent ATP4 transporter, and were acquired by exposing parasites to sub-lethal concentrations of a spiroindolone [18] , an aminopyrazole [19] , or other scaffolds from the Tres Cantos Antimalarial Set library [20] . These two resistance genes were represented by multiple strains since critical SNV mutations may be located within an active site or result in a change in membrane potential, resulting in each mutation only affecting a subset of PfATP4 or cytochrome bc1 inhibitors. To evaluate potential overlapping activity against known antimalarial drug targets, we performed dose-response studies with each compound against our assembled set of drug-resistant lines and their corresponding parents, in an asexual blood stage proliferation assay ( Table 1 ). Comparisons were made to the drug-sensitive strain 3D7 when a parent was unavailable (TM90C2A, W2 and Dd2). As laboratories conducted EC 50 assays with different strains and protocols, all comparisons were made between assays from the same laboratory and under the same assay conditions. Compounds displaying >5-fold EC 50 shifts relative to the parent or sensitive strain were flagged as having potentially non-novel targets. Average fold shifts per strain ranged from 0.82 to 2.34, with a median of 1.23 indicating there was not common resistance to any one resistant clone. No resistance patterns were observed when classifying the compounds based on chemical structure, but this was not surprising given the diversity of compounds chosen. On the other hand, given that these confirmed compounds were derived from larger unconfirmed hit lists to which some filtration criteria may have been applied (for example, elimination of obvious dihydrofolate reductase inhibitors [32] ), some [10] , [11] , [12] , [13] pre-existing bias may exist in the set. Table 1 Summary of mutated strains testing cross-resistance Full size table Alleles in the strain set generally did not confer resistance to the vast majority of the compounds ( Fig. 2a ), with only two compounds (MMV019066 and MMV008149) losing efficacy in some resistant lines relative to their parent clones (EC 50 fold-shifts >5-fold). ATQ-R4, bearing a Q o cytochrome bc 1 allele, was resistant to a propanamide, MMV019066, ( P value=0.0016) with an EC 50 fold-shift of 16 × , as determined by a one-way analysis of variance (ANOVA) analysis with a Dunnett’s multiple comparison correction. In addition, CYTb-G131S, a cytochrome bc 1 Q o allele, demonstrated complete resistance to MMV008149, a carboxamide, with a >38-fold change in EC 50 . Statistically significant resistance was seen against MMV019066 and MMV008149 in other cytochrome bc 1 Q o mutants (ATQ-R5 and ATQ-R4, respectively), but the EC 50 fold-shifts seen were under the threshold value set for the study. Neither compound shared any structural features with other cytochrome bc 1 inhibitors, including atovaquone and decoquinate ( Fig. 2b ). 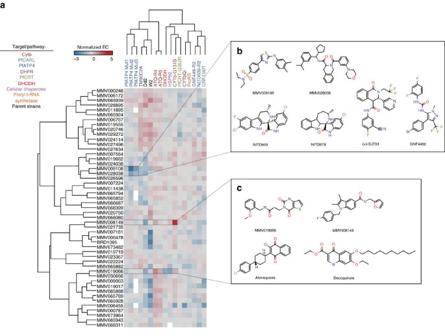Figure 2: Cross-resistance fold shifts observed in compound set. (a) A total of 15 resistant strains were tested with each MMV compound to identify potential pre-existing cross-resistance. Calculating the fold shifts between each clone and either a corresponding parent or a drug sensitive 3D7 strain generated the heatmap. To normalize conferred resistance and sensitivity, the natural log of each fold shift is displayed. Fold shifts instead of raw data were used as multiple assays were run with varying times and detection indicators. Incomplete cross-resistance assays are depicted in white. All assays were run in triplicate. For one compound (BRD1095), a close analogue (BRD3444) was analysed for TM90C2A and PfATP4-Mut1–3. SMILEs for all compounds are listed inSupplementary Data 1. (b) Chemical structures of the two MMV compounds (MMV009108 and MMV028038) with increased efficacy against one or morepfatp4mutated clones. Both compounds displayed low structural similarity to a number of other knownpfatp4inhibitors. (c) Chemical structures of the two MMV compounds (MMV019066 and MMV008149) with decreased efficacy against one or more cytochromebc1mutated clones. Atovaquone and decoquinate, two other cytochromebc1inhibitors, were structurally significantly different. Figure 2: Cross-resistance fold shifts observed in compound set. ( a ) A total of 15 resistant strains were tested with each MMV compound to identify potential pre-existing cross-resistance. Calculating the fold shifts between each clone and either a corresponding parent or a drug sensitive 3D7 strain generated the heatmap. To normalize conferred resistance and sensitivity, the natural log of each fold shift is displayed. Fold shifts instead of raw data were used as multiple assays were run with varying times and detection indicators. Incomplete cross-resistance assays are depicted in white. All assays were run in triplicate. For one compound (BRD1095), a close analogue (BRD3444) was analysed for TM90C2A and PfATP4-Mut1–3. SMILEs for all compounds are listed in Supplementary Data 1 . ( b ) Chemical structures of the two MMV compounds (MMV009108 and MMV028038) with increased efficacy against one or more pfatp4 mutated clones. Both compounds displayed low structural similarity to a number of other known pfatp4 inhibitors. ( c ) Chemical structures of the two MMV compounds (MMV019066 and MMV008149) with decreased efficacy against one or more cytochrome bc1 mutated clones. Atovaquone and decoquinate, two other cytochrome bc1 inhibitors, were structurally significantly different. Full size image As had been previously observed [19] , mutations in PfATP4 resulted in parasites that were more sensitive to unrelated compounds: ATP4-Mut2 exhibited sensitivity to a sulfonamide (MMV009108— P value=0.0001; 23 × fold-shift) and a carboxamide (MMV028038— P value=0.0007; 5 × fold-shift). ATP4-Mut3 additionally conferred sensitivity to MMV009108 ( P value=0.0047; 5.2 × fold-shift). Neither compound was structurally similar to spiroindolones, pyrazoles or dihydroisoquinolones, all previously identified PfATP4 inhibitors (NITD609 (ref. 18 ), KAE678 (ref. 18 ), GNF4492 (ref. 19 ) and (+)-SJ733 (ref. 20 )), with a Tanimoto coefficient range of 0.127–0.34 ( Fig. 2c ). Finally, two compounds (MMV665939 and MMV028895) lost efficacy in the parent strains W2 or Dd2 when compared with the 3D7 sensitive strain within the same lab. MMV665939 demonstrated fold shifts in W2 compared with 3D7 (EC 50 fold-shift—9.5 ×), as well as in the other two W2-based clones (PfATP4-Mut1: 16.6 × , PfATP4-Mut2: 18.9 ×) compared with 3D7. Fold shifts in Dd2 compared with 3D7 were also seen in MMV665939, though these shifts were less severe (1.5–3.1 × ; average 2.4 ×). MMV028895 showed reduced efficacy in Dd2 (EC 50 fold-shift 7.1 ×), which was also seen throughout the other Dd2 clones (2.0–7.5 × ; average—5.5 ×), but unlike MMV665939 maintained potency against W2 strains. These efficacy changes in Dd2 and W2 are most likely due to pfmdr , given that W2 and Dd2 contain additional copies of the multi-drug resistance gene (2 and 3–4 copies, respectively) when compared to 3D7. Selection of resistant parasites While we found an overall lack of pre-existing resistance, analysing the onset of resistance was critical, as compounds resulting in rapid resistance are not ideal for clinical development. We therefore sought to create drug-resistant parasites using a variety of different selection methods. We implemented either a high-dose method or a ramp-up/pulse method for our in vitro selections. Two of the 50 compounds—MMV028895 and MMV665824—were removed from the selection study during experimentation. MMV665824 was removed due to a significant loss of potency, while MMV028895 exhibited cross-resistance to resistant parasites generated by MMV007564. Out of the remaining 48 compounds, resistant parasites were obtained for 23 ( Supplementary Data 1 ). As each selection was performed in triplicate with three independent cultures, we succeeded in generating a total of 66 resistant cultures. Parasites resistant to MMV026596 were not obtained despite 100 days of selection, but the cultures acquired hypersensitivity to mefloquine with a 10-fold reduction in EC 50 compared with its parental line, 3D7. For the remaining 24 compounds, acquisition of resistant parasites was unsuccessful despite numerous attempts over an extensive period of time. To determine if the cross-resistance assay was predictive, we sought to determine the target of MMV008149, the compound resulting in the largest EC 50 fold-shift (>38 ×) within the cross-resistance assay set by fully sequencing six parasite clones that had acquired resistance to MMV008149. The EC 50 values for the resistant lines ranged from 1.67 μM to 10.06 μM, a 3–21 × EC 50 -fold change when compared with the Dd2 parent (EC 50 =485 nM). Genomic DNA (gDNA) was isolated from the Dd2 parent and six clones (two clones per resistant selection flask), and samples were prepared for whole-genome sequencing. Samples were sequenced to >60 × coverage using paired end reads and aligned to the 3D7 reference genome and variants were called with HaplotypeCaller (GATK). Comparing the nucleotide variation found in the resistant samples to the Dd2 parent clone, which had been isolated immediately before selections, we identified genomic changes that had presumably occurred during selection. Following this comparison, 19 mutations were identified: 11 SNVs and eight insertion/deletions (INDELs) ( Table 2 , Supplementary Data 2 ). INDEL mutations were comprised of intergenic (three), codon INDEL (three), intronic (one) and frame-shift (one) mutations. The SNV set showed a mixture of intergenic (five), synonymous (three) and non-synonymous (three) mutations. Comparing all six clones, one gene was mutated across all samples: cytochrome bc1 . Additionally, variant positions correlated well to EC 50 fold changes, with the lower fold changes (3.4–5.9 ×) corresponding to the G131S amino acid change, and the higher EC 50 fold-shifts (18–21 ×) corresponding to the Y126C and V284L amino acid changes. Two of the mutations, G131S and Y126C, were contained in the Q o site, while the third mutation (V284L) was not in either the Q o or Q i binding region [29] . G131S was also the major mutation found in CYTb-G131S, the cross-resistant strain predicting cytochrome bc1 as a potential target for MMV008149. These results support that the cross-resistance assay was able to successfully identify compounds with overlapping targets, and made us more confident that our compound set consisted of novel targets. Table 2 SNV and INDEL mutations in MMV008149 Full size table Multi-stage activity profiling As drugs that eliminate multiple stages of the parasite lifecycle will be critical components in global efforts to eliminate malaria [10] , we were interested in knowing whether the compounds in our study had additional activities against either the liver and/or transmission stages of the parasite lifecycle. To determine this, we first evaluated the compounds in additional phenotypic assays. The first assay was a P. berghei hepatocyte invasion and development assay, which predicts causal prophylactic activity. Hepatocyte toxicity was additionally tested to identify false-positive activity in the liver stage due to host-cell toxicity. Assays were executed in duplicate using a 12-point EC 50 curve at starting concentrations of 5 μM or 50 μM ( Supplementary Table 1 ). Positive and negative controls testing for hepatocyte toxicity and liver stage activity included atovaquone (PfLuc EC 50 :0.419±0.044 nM; HepG2 EC 50 :7720±1370, nM) and puromycin (PfLuc EC 50 :32.7±29.7 nM; HepG2 EC 50 :254±36.6 nM). Of the 47 compounds examined, 15 were found to be active against liver-stage parasites (EC 50 values <1 μM (10–880 nM)), nine of which demonstrated a minimal fivefold difference between parasite activity and hepatocyte toxicity ( Supplementary Fig. 1 ). Interestingly, six compounds were more potent in the liver stage than in the asexual stage. The most significant potency change was seen with MMV019066, a propanamide, which had a reduction in EC 50 from 1.67 μM to 0.31 μM and previously demonstrated cross-resistance with cytochrome bc 1 alleles. This was expected given that cytochrome bc 1 inhibitors are highly active against liver stages. MMV024038, a quinoline sulfonamide, also demonstrated a reduction in EC 50 from 228 nM to 10 nM. This compound, however, exhibited some hepatocyte toxicity (146 nM); thus the indirect effects of the host-cell environment on parasite growth could not be ruled out. The second assay was a late-stage (stage V) gametocyte survival assay, which predicts transmission-blocking activity. Assays were executed in duplicate using a 12-point EC 50 curve at starting concentrations of 1.25 μM or 12.5 μM ( Supplementary Table 1 ). Positive and negative control compounds included puromycin (0.61±0.11 μM) and atovaquone (> 12.50 μM), respectively. For the late-stage gametocyte assay, 12 compounds resulted in EC 50 values <1 μM (260–990 nM), 50% of which overlap with the 15 compounds found to have activity in the liver-stage assay. Of the six compounds with complete multi-stage activity, 83% (5/6) demonstrated hepatocyte toxicity >10 × the liver stage EC 50 . Unlike the liver stage, none of the compounds had increased potency against sexual stage compared with the asexual parasites, which was expected as previous literature has found that most currently used antimalarials yield higher EC 50 values against late-stage gametocytes when compared with the asexual stage EC 50 (ref. 13 ). Five compounds, however, demonstrated late-stage gametocyte EC 50 values within a twofold range of the asexual EC 50 value. Rate of killing assays To identify whether selection success could be predicted by compound speed of action, and to gain a greater insight into the potential mechanisms of action, assays were performed to test the killing rate ( Supplementary Data 1 ) [33] . To quantify the killing rate, viability time-course profiles for each compound were compared with antimalarials known to have fast (chloroquine), moderate (pyrimethamine) or slow (atovaquone) rate of action. These rates were then compared with other compound characteristics, including cross-resistance profile, selection success, potency and structural characteristics to identify any possible trends. Overall, the compound set resulted in a fairly even distribution of fast, moderate and slow speeds ( Fig. 3a ), implying there was no bias in the phenotypic screens for a particular killing rate. One compound’s rate of killing, MMV666080, was unidentifiable due to compound availability. No correlation was seen between compound structure and speed of action. Additionally, there was no correlation found between killing rate and compound potency against 3D7, nor between potency and selection success ( Supplementary Fig. 2 ). 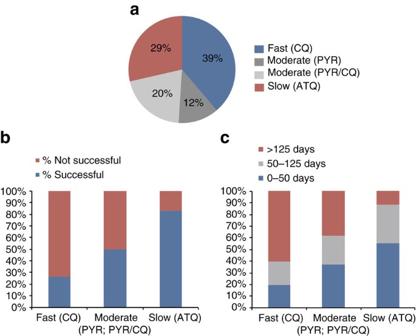Figure 3: Killing rate trends. (a) Proportion of fast (CQ), moderate (PYR or PYR/CQ), and slow (ATQ) compound killing rates in our compound set (49 compounds in analysis). (b) Proportion of failed and successful compound selections sorted by killing rate (47 compounds in analysis). (c) Successful selections further proportioned out based on amount of time required to result in resistant parasites. Trend in selection success and killing rate was found to be statistically significant (P=0.0022) by a one-tailed Fisher’s exact test. Figure 3: Killing rate trends. ( a ) Proportion of fast (CQ), moderate (PYR or PYR/CQ), and slow (ATQ) compound killing rates in our compound set (49 compounds in analysis). ( b ) Proportion of failed and successful compound selections sorted by killing rate (47 compounds in analysis). ( c ) Successful selections further proportioned out based on amount of time required to result in resistant parasites. Trend in selection success and killing rate was found to be statistically significant ( P =0.0022) by a one-tailed Fisher’s exact test. Full size image Comparing the selection success rate to compound rate of killing, we saw a significant positive correlation ( P =0.0022) between speeds of action and selection success, as determined by a one-tailed Fisher’s exact test. ( Fig. 3b,c ). Of the 12 selections with compounds demonstrating a slow speed of action, 83% (10/12) were successful. This was in contrast to compounds with fast-killing rates of which only 26% (5/19) were successful. Additionally, within each set of successful selections, we noticed a trend within the length of time to generate resistant parasites. For the fast-acting compounds, 3/5 successful selections took >125 days, whereas 5/10 resistant parasites were successfully selected for within 50 days for slow-acting compounds. Therefore, slower compounds typically had greater success and required shorter periods of time to develop resistance when compared with fast-acting compounds. This trend remained relatively consistent within individual labs. These results confirm previous findings of faster acting compounds having a lower propensity for developing de novo resistance [34] . Fast-acting compounds are already desirable in the clinic due to a quick clearance of parasites and alleviation of symptoms, as well as their propensity towards slower drug resistance development. The inability to develop resistance in vitro , however, even when using slow ramp-up selection methods may imply that these benefits come from the target itself. These genes may have minimal mutational flexibility or inhibitors may target several genes, making them ideal for exploitation in antimalarial development. Alternatively, some compounds may have human host targets instead of parasite targets and affect the erythrocyte directly. Further work is required to distinguish between these possibilities. Every therapeutic, whether for the treatment of infectious agents or malignant tumours, is in a race against time; a race against the inevitable development of drug resistance leading to reduced clinical effectiveness. Many factors play a role in the development of resistance, from evolutionary and biochemical constraints of the targeted organism to therapy regimens and the overuse or misuse of therapeutics. Not all therapeutics, however, are created equal. A detailed understanding of a targeted organism’s biology and the critical factors required to minimize the emergence of resistance provide opportunities to design more effective and long-lasting drugs and drug combinations. This requires an extensive knowledge of the organism, as well as a comprehensive understanding of how resistance evolves. This study represents the first systematic analysis of cross-resistance in malaria parasites. We have assessed 50 antimalarial compounds with diverse chemical structures, rates of parasite killing and stage specificity. With few exceptions, the compounds studied did not demonstrate significant cross-resistance to previously identified targets, indicating a large potential to identify additional druggable pathways in the parasite and further our arsenal of antimalarial therapeutics. A lack of cross-resistance to known drug targets does not mean that resistance will not quickly develop, however, and the resistance ‘life expectancy’ and resulting fitness costs need to be considered for any potential clinical candidate. In selecting for resistant mutants, we found that fast-acting compounds are harder to develop resistance against and generally have a longer onset of resistance when compared with slow-acting compounds. Given that compound killing rates are thought to be determined primarily by their mode-of-action, this resistance feature may be largely due the target or targets themselves. Moving forward, it will be important to verify if this trend holds in compounds with multi-stage activity, as only a small fraction of our compounds (6/50) demonstrated activity against asexual, sexual and liver stage parasites, and multi-stage active antimalarials will be vital in achieving malarial elimination. In addition to killing rate, our compound set provides a list of various physicochemical and structural features that may additionally be predictive of selection success, and the addition of our set to future screens may provide an eventual predictive model, focusing on compounds less likely to be prone to resistance development ( Supplementary Figs 3 and 4 ). Fast-acting compounds have already been a focus in therapeutic development as they rapidly stop disease progression and avoid severe complications, but the additional benefit of reduced evolution of resistance makes them even more attractive candidates for future antimalarial designs. Compound origin and computational clustering Compounds were all publically available and obtained from a variety of sources, including the medicines for malaria venture (MMV) malaria box [10] , the GlaxoSmithKline Tres Cantos Antimalarial Set [11] , the University of Dundee and the Broad Institute’s Diversity Oriented Synthesis libraries, as indicated in Supplementary Data 1 . Compound similarity was calculated using the flexible MCS (FMCS) finder package in R. Clustering was conducted using hclust with a ward.D2 method setting. Pairwise distances were calculated between Tanimoto coefficient values from fmcsR. Strain culture origins and propagation P. falciparum parent strains 3D7 and Dd2 used for selection were obtained from the labs of Dan Goldberg and David Fidock, respectively. The Fidock lab additionally supplied the Dd2Δexo strain for selections with MMV000787 and MMV023367. Functional assay and cross-resistant strains were obtained from the labs of Elizabeth Winzeler, Dyann Wirth, David Fidock and GlaxoSmithKline, as listed in Table 1 . Asexual parasites were grown with 5% haematocrit at 37 °C in RPMI (Rosewell Park Memorial Institute)-1640 medium supplemented with 0.014 mg ml −1 hypoxanthine, 38.4 mM HEPES, 0.2% NaHCO 3 , 0.2% glucose, 3.4 mM NaOH, 0.3 g l −1 glutamine and 5% AlbuMAX II. Depending on lab preferences, parasites were grown either in the presence or absence of 0.05 mg ml −1 gentamicin and 4.2% human O + serum (Interstate Blood Bank, Inc.). Cultures were maintained in a gas mixture of 5% O 2 , 5% CO 2 and 90% N 2 . When not undergoing selections, cultures were maintained with media changes every other day, keeping parasitemia values at 0.3–4%. Frozen stocks were prepared using one of two methods: (1) by freezing 100% red blood cells (RBCs) at ∼ 5% parasitemia with equal volumes of a freezing solution composed of 28% glycerol, 3% sorbitol and 0.65% NaCl; (2) freezing 0.2 ml RBCs at ∼ 5% parasitemia with 0.3 ml serum and 0.5 ml of a glycerol solution. Stocks were thawed out by slowly adding 1/5 volume of 12% NaCl, followed by five volumes of 1.6% NaCl. Parasites were then spun down at 800 g for 5 min at room temperature and washed with supplemented media before standard culturing methods. Cross-resistance and functional assays EC 50 assays were conducted using either a 48 or 72-h assay based on lab preference and specialty (internal assay variance summarized in Supplementary Fig. 5 ). The 48-h assay was carried out in a 96-well format following standard methods using the 3 H-hypoxanthine incorporation assay [35] . The raw EC50 values corresponding to this assay can be found in Supplementary Data 3 . Briefly, this assay relies on the parasite incorporation of labelled hypoxanthine that is proportional to P. falciparum growth. A culture of parasitized RBCs (0.5% parasitemia with a percentage of ring stage higher than 70% of total parasitemia, 2.0% haematocrit) in RPMI-1640, 5% AlbuMAX and 5 μM hypoxanthine was exposed to drug serial dilutions. Plates were incubated for 24 h at 37 °C, 5% CO 2 , 5% O 2 and 90% N 2 . After 24 h of incubation, 3 H-hypoxanthine was added and plates were incubated for an additional 24-h period. After that, parasites were harvested on a glass fibre filter using a TOMTEC Cell Harvester 96. Filters were dried and melt-on scintillator sheets were used to determine the incorporation of 3 H-hypoxanthine. Radioactivity was measured using a microbeta counter. Data were normalized using the incorporation of the positive (parasitized RBCs without drug) and negative (same culture with artesunate at 2 μM) controls. All assays were conducted in triplicate using three independently grown cultures, and EC 50 values were determined using the XLfit add-in module for Excel (version 2.3.1) from Grafit (version 5.3.1.3), where parameter h is the assay hill slope, x is the compound concentration and y is the inhibition of growth effect. The XLfit equation is: Additionally, any EC 50 outliers were removed using a single iteration of Grubbs’ test, eliminating values with z -scores above the critical z- value ( α =0.05). Alternatively, a SYBR Green-based proliferation approach was used for the 72-h assay, as previously described [32] . Briefly, a culture of either synchronized or asynchronous parasitized RBCs (0.3% parasitemia and 4% haematocrit) in screening medium (identical to supplemented medium above except no serum was added) was exposed to serial drug dilutions. Plates were incubated at 37 °C and gassed with 93% N2, 4% CO2 and 3% O2 for 72 h. Following incubation, 10 × SYBR Green I (Invitrogen; supplied in 10,000 × concentration) in lysis buffer (20 nM Tris-HCL, 5 mM EDTA, 0.16% Saponin wt per vol and 1.6% Triton X vol per vol) was added to the wells and the plates were incubated overnight at room temperature before plate reading. EC 50 assays were repeated three times, taking the average EC 50 value from each assay set, and removing any outliers using a single iteration of Grubbs’ test, eliminating values with z -scores above the critical z -value ( α =0.05). The raw EC50 values for synchronized parasites assayed in a 384-well format are listed in Supplementary Data 4 . The raw EC50 values for asynchronous parasites assayed in a 96 or 1536-well format are listed in Supplementary Data 5 . EC 50 values for each strain were compared with those of the corresponding parent strain to determine fold-shift changes and identify resistance. To minimize the cause variance between assays, all comparisons were conducted between strains assayed under identical conditions. A one-way ANOVA followed by a Dunnet’s post-test was conducted in GraphPad Prism to identify significant changes between the parent and resistant strain. For the purposes of this study and to minimize false positive, compounds displaying >5-fold EC 50 shifts and determined to be significantly different from its corresponding parent by a one-way ANOVA analysis were identified as having potentially non-novel targets. Cross-resistance computational analysis Computational analysis of cross-resistance was conducted in R. Briefly, EC 50 fold shift ratios were calculated using log transformed EC 50 values from the parental and resistant strains. As EC 50 assays were run across multiple labs, any strain fold-shift calculations were conducted between strains run within the same lab to minimize error due to assay variability. The natural log of the ratios was loaded into R, and a heatmap analysis was executed using heatmap.2 from the gplots package. Compounds were clustered by structural similarity (fmcsR) and strains were clustered by column mean values. Evolution of compound-resistant lines Based on the compound speed of action and lab specialty, selections were conducted using a high-pressure intermittent selection method, a step-wise selection method, or a constant selection method. For high-pressure selections, ∼ 1–2 × 10 9 parasites were treated at a concentration of 3–10 × EC 50 until parasites could not be seen by microscopy (4–10 days). Following treatment, compound pressure was removed and cultures were allowed to recover. Once healthy parasites were seen and parasitemia reached ∼ 2%, compound pressure was reinstated. For step-wise selections, ∼ 1 × 10 8 parasites were treated at a starting concentration resulting in a reduced growth rate of 50%. Cultures were examined daily by microscopy, increasing compound concentration in increments of 5–10% as needed to maintain a 50% reduced growth rate. Selections were carried out until cultures achieved a reproducible EC 50 fold shift of >3 × . Finally, constant selections were conducted in a similar manner to the high-pressure intermittent method with the exception that compound pressure was never removed. Following successful selection, cultures were cloned out using a limiting dilution method as previously described [36] . Selections were terminated after 200 days if resistance could not be obtained. Library preparation and analysis of sequenced samples gDNA was obtained from parasites by washing infected RBCs with 0.05% saponin and isolating the gDNA using a DNeasy Blood and Tissue Kit (Qiagen), following the standard protocols. To prepare the sequencing libraries, gDNA was tagmented and amplified with the Nextera XT kit (Cat. No FC-131–1024, Illumina) using the standard dual index protocol, and sequenced on the Illumina HiSeq 2500 with a RapidRun mode, sequencing 100 base pairs deep on either end of the fragments. Following sequencing, reads were aligned to the P. falciparum 3D7 reference genome (PlasmoDB v. 13.0), following the Platypus pipeline as previously described, with the exception that SNVs and INDELs were called with GATK’s HaplotypeCaller [37] . To identify valid variants, mutations were filtered using general recommendations from GATK ( Supplementary Table 2 ). Following the initial filtration, mutations where read coverage were <5 and/or where mixed read ratios were>0.2 (reference/total reads) across all samples were removed. Rate of killing and multi-stage activity assays Rate of killing was determined for each compound following a previously described methodology, which uses the invasion of fresh erythrocytes as surrogate of parasite viability [33] . Briefly, parasites were treated with compounds for 48 h. Compound was washed out and fresh-labelled erythrocytes added to the treated parasites. Double stained erythrocytes (RBC label plus parasite DNA label) were quantified and per cent of survival determined. Liver-stage activity was determined by pretreating hepatic human cells (HepG2) for 2 h with compound in 1,536-well plates infected with freshly dissected P. berghei sporozoites. After 48 h of incubation, the viability of P. berghei exoerythrocytic forms was measured by luminescence reaction light output using BrightGlo (Promega). Varying levels of compound concentration were used (5 μM or 50 μM) due to the stock concentration supplied. To test sexual-stage activity, compounds were tested against late-stage gametocytes using a MitoTracker fluorescent-based assay [13] . Specifically, synchronized stage V gametocytes were incubated with compound for 72 h. MitoTracker Red CMXRos (Life Technologies) was added to each well (final concentration: 500 nM) together with saponin to lyse the RBCs. Each plate was then imaged with an Operetta High Content Imaging System (Perkin Elmer) for fluorescence (590–640 nm). Varying levels of compound concentration were used (1.25 μM or 12.5 μM) due to the stock concentration supplied. The gametocytocidal activity was measured using high-content image analysis software (Harmony, Perkin Elmer). The readout was based on number of metabolically active gametocytes per well. Cheminformatics predictors We evaluated the association between acquisition of drug resistance and pharmacological, physicochemical and structural characteristics of the 48 compounds for which selection was attempted. Specifically, we considered the following properties: (1) pharmacological properties measured in this study: killing rate, toxicity and EC 50 at three different stages of parasite development; (2) 51 physicochemical descriptors obtained with QikProp software [38] and 129 descriptors obtained with VolSurf+ (ref. 39 ); and (3) 2,694 extended-connectivity fingerprints that encode circular substructures with a bond diameter of 10, generated by ChemAxon software (ChemAxon, Kft.) [40] ; and (4) 194 hierarchical scaffolds associated with the compounds generated by HierS software [41] . For each feature, we measured statistical significance of its relationship to the selection success, taking into account the nature of the features [42] . In particular, structural features (that is, extended-connectivity fingerprints and scaffolds) are binary and indicate the presence or absence of each structural element in a compound. For these reasons, hypergeometric statistical tests were applied to structural features and t -tests were applied to pharmacological and physiochemical features to measure statistical significance. Data availability All 66 resistant P. falciparum lines will be deposited to the Malaria Research and Reference Reagent Resource Center (MR4) and will be made available on request to E.A.W. All relevant sequence data have been deposited in the National Center for Biotechnology Information (NCBI) Sequence Read Archive database with accession code SRP069308. The authors declare that all other data supporting the findings of this study are available within the article and its Supplementary Information files. Accession codes : All relevant sequence data have been deposited in the National Center for Biotechnology Information (NCBI) Sequence Read Archive database with accession code SRP069308. How to cite this article : Corey, V. C. et al. A broad analysis of resistance development in the malaria parasite. Nat. Commun. 7:11901 doi: 10.1038/ncomms11901 (2016).